Hybrid superconducting-magnetic memory device using competing order parameters In a hybrid superconducting-magnetic device, two order parameters compete, with one type of order suppressing the other. Recent interest in ultra-low-power, high-density cryogenic memories has spurred new efforts to simultaneously exploit superconducting and magnetic properties so as to create novel switching elements having these two competing orders. Here we describe a reconfigurable two-layer magnetic spin valve integrated within a Josephson junction. Our measurements separate the suppression in the superconducting coupling due to the exchange field in the magnetic layers, which causes depairing of the supercurrent, from the suppression due to the stray magnetic field. The exchange field suppression of the superconducting order parameter is a tunable and switchable behaviour that is also scalable to nanometer device dimensions. These devices demonstrate non-volatile, size-independent switching of Josephson coupling, in magnitude as well as phase, and they may enable practical nanoscale superconducting memory devices. Superconducting and magnetic devices have a long but mutually exclusive history due to the fact that the order parameters are competing, magnetic order suppresses superconducting order and vice versa. Superconducting Josephson junctions (JJs), which rely on modulating the magnitude and phase of the superconducting order parameter , have been developed for microwave oscillators, voltage standards, logic gates and sensitive magnetic field detectors [1] . Magnetic devices, which rely on manipulating the local magnetization , have been developed for magnetic random access memory, field sensors for recording heads and high frequency spin-transfer oscillators [2] , [3] . Recent advances in the understanding of superconductor–ferromagnet (S–F) hybrid structures have revealed exciting physical phenomena, such as devices in which the Josephson ground-state phase difference between the two superconductors is shifted by π compared with that of conventional junctions, or in which Josephson coupling is achieved via spin-polarized triplet states [4] , [5] . Combining the superconducting quantum and spintronic effects into low-power bi-stable devices that are switchable between different memory states could transform high-performance computing and elevate superconducting digital technology [6] as a serious alternative to existing power-hungry computers based on semiconductor technology. Despite the demonstration, over a decade ago, of an ≈700 GHz clock-rate RSFQ (rapid single flux quantum) logic element [7] , the lack of a practical and scalable cryogenic memory is one reason that superconducting digital electronics has been implemented only in niche applications [8] , [9] . Past cryogenic-memory efforts employed circuits that stored magnetic flux quanta in superconducting loops or combined Josephson and complementary metal–oxide–semiconductor technologies in hybrid circuits [10] , [11] . Unfortunately, these approaches did not simultaneously offer high speed, ultra-low power and scalability. Storing information within a JJ by changing its state is a straightforward approach to making a cryogenic memory that is both practical and scalable. One way to do this is by inserting magnetic layers within the barrier of a JJ so that the magnetic configuration changes the superconducting critical current that separates zero and non-zero voltage states [12] , [13] , [14] , [15] . A number of magnetically controlled Josephson switches have been demonstrated. Clinton and Johnson [16] demonstrated microbridge devices that switched between different critical currents using the stray field of a ferromagnet. More recently, critical-current switching was demonstrated by incorporating a single ferromagnetic layer into a JJ barrier [13] . In both devices, the difference in the critical current of the two states, or the signal contrast, comes from the magnitude and direction of the remanent magnetic field within the microbridge or the junction barrier. However, these devices will require a significant ferromagnetic moment and, thus, a high magnetic switching energy at submicrometer junction dimensions, which would make them practical only for low-density memory. Scalable JJ devices should be based on direct manipulation of the Josephson coupling instead of a field effect. Although triplet superconductivity in S–F structures has recently become a subject of intense study due to the finite spin current and the long Cooper-pair coherence length in a ferromagnet [5] , [17] , and they may be useful as memory devices, we focus on JJs based on pseudo-spin-valve (PSV) barriers and spin-singlet pair states because of their simpler physical and conceptual structure. A PSV comprises two different ferromagnetic layers separated by a non-magnetic metal. Typically, its resistance state is changed through the giant magnetoresistance (GMR) effect by changing the orientation of the magnetization of one layer with respect to the other [2] . Writing information (that is, switching the PSV state between the parallel (P) and anti-parallel (AP) magnetizations) to a typical PSV device can be accomplished either by applying a magnetic field to switch the magnetization of the layer with lower coercivity or, in nanoscale devices, by applying a bias current to switch the magnetization through the spin-transfer torque effect [18] . Regarding the superconducting transport properties of an S–PSV–S JJ, S–F proximity theory provides the basic physical understanding [4] , [5] . The exchange field in the ferromagnet splits the two electronic spin bands, resulting in a spatial phase modulation of the Cooper-pair condensate emanating from each superconductor. This effect leads to oscillating decay, including sign reversal, of the Josephson coupling as a function of the magnetic barrier thickness. By placing a second F layer in the barrier, the total phase shift may be increased or decreased, depending on the relative orientations of the magnetizations of the F layers (that is, P or AP), and this may produce a corresponding change in the critical current of the junction [19] , [20] , [21] . Experimental studies of JJs with double magnetic barriers of collinear magnetizations were carried out by Bell et al. [12] and later by Robinson et al. [22] In both studies, enhanced maximum supercurrents were observed for the AP states compared with the P states. Both works concluded that their results were due to the exchange-field effect on the pair phase, based on an argument that the phase shift in the AP state was smaller than in the P state and produced a larger, less-modulated critical current. However, the interpretation of these results is complicated by competing effects. In such structures, a remanent field from the magnetic barrier induces a non-uniform supercurrent distribution within the junction and results in a maximum total supercurrent I m that is reduced from the critical current I c ≡ J c A , given by critical current density J c and the junction area A (refs 23 , 24 ). The higher I m in the AP state may be attributed to the lower average remanent field, as compared with that of the P state. Thus, to fully characterize the state of such a junction, we must extract the I c , which is the maximum supercurrent at zero net flux in the barrier (not at zero applied field), determined from the maximum value of I m ( H ), where H is the applied magnetic field. In this work, we perform detailed I m ( H ) and other measurements to clearly discriminate between the remanent-field effect and the more direct exchange-field effect on Josephson coupling. Distinguishing these two effects is key to understanding the physics governing these devices and evaluating their scaling potential. We show well-controlled changes in Josephson coupling in amplitude or in phase by carefully selecting magnetic barrier thicknesses. Device development and characterization We find that the material choices are crucial in obtaining unambiguous results. The PSV must include materials with different coercivities so that the device can be placed into both the P and AP states. Weaker ferromagnets make the oscillation and decay length of the Cooper pair longer and enable the use of thicker films, which is advantageous for the reproducibility of the devices. However, the free-layer coercivity must be high enough to show a large portion, including the peak, of the main lobe of the Fraunhofer pattern associated with each magnetic state of the PSV. We used Ni as the higher-coercivity layer, as its saturation magnetization is relatively low, and at 10 K its measured coercivity is ≈40 mT, which is adequate for a PSV hard layer. For the free layer, we chose Ni 0.7 Fe 0.17 Nb 0.13 , which had a coercivity of ≈2 mT at 10 K and a reduced magnetic moment with Nb doping [25] ( Fig. 1 , inset). The S–PSV–S multilayer films were sputter-deposited on oxidized silicon wafers in a chamber without breaking vacuum. Each device had the following film deposition sequence and thicknesses: Nb(100 nm)/Cu(3 nm)/Ni 0.7 Fe 0.17 Nb 0.13 ( d NiFeNb )/Cu(5 nm)/Ni( d Ni )/Cu(3 nm)/Nb(70 nm). The Ni 0.7 Fe 0.17 Nb 0.13 layers were grown by co-sputtering Ni 0.8 Fe 0.2 and Nb targets. The Cu layers adjacent to each Nb layer serve as buffers or growth templates for the ferromagnetic layers and are expected to be superconducting due to the proximity effect at 4 K. The centre spacer Cu layer prevents exchange coupling and reduces magnetostatic coupling between the Ni 0.7 Fe 0.17 Nb 0.13 and the Ni, allowing them to switch independently. Using a superconducting quantum interference device magnetometer, we measured the Nb superconducting temperature T c ≈8.9 K and observed hysteretic magnetization loops with two well-separated switching fields in the unpatterned multilayers ( Fig. 1 ). 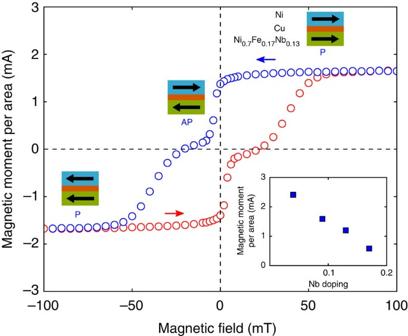Figure 1: Hysteretic magnetization data from an unpatterned PSV multilayer structure. The multilayer structure is Nb(100 nm)/Cu(3 nm)/Ni0.7Fe0.17Nb0.13(2.1 nm)/Cu(5 nm)/Ni(3 nm)/Cu(3 nm)/Nb(70 nm). The measurement temperature is 10 K. The field was swept from positive to negative (blue circles), then back to positive (red circles), as indicated by the coloured arrows. Illustrated above the plot are the different magnetization states (P: parallel; AP: antiparallel) of the Ni and Ni0.7Fe0.17Nb0.13for the trace with the blue circles. Inset: Trend of Ni0.7Fe0.17Nb0.13saturation magnetization with Nb doping. Figure 1: Hysteretic magnetization data from an unpatterned PSV multilayer structure. The multilayer structure is Nb(100 nm)/Cu(3 nm)/Ni 0.7 Fe 0.17 Nb 0.13 (2.1 nm)/Cu(5 nm)/Ni(3 nm)/Cu(3 nm)/Nb(70 nm). The measurement temperature is 10 K. The field was swept from positive to negative (blue circles), then back to positive (red circles), as indicated by the coloured arrows. Illustrated above the plot are the different magnetization states (P: parallel; AP: antiparallel) of the Ni and Ni 0.7 Fe 0.17 Nb 0.13 for the trace with the blue circles. Inset: Trend of Ni 0.7 Fe 0.17 Nb 0.13 saturation magnetization with Nb doping. Full size image Four-point electrical measurements were used to characterize JJs with different dimensions and barrier materials. Wafers of test chips containing these junctions were fabricated with reliable, high-throughput processes, employing stepper lithography and reactive ion etching. The barrier etching was done by ion milling monitored with an ion mass spectrometer. The rest of the fabrication process is similar to that used to fabricate NIST Josephson voltage standards [26] . There was no noticeable deleterious change in the magnetic properties of the films due to the device processing. For junctions with designed dimensions <2 μm, the actual fabricated feature dimensions were significantly smaller due to process runout (the difference between the design and actual dimensions). For example, the smallest junctions studied were elliptical, with the short and long axes of 0.9 μm and 1.8 μm, respectively, by design, but yielded effective areas A eff ≈0.5 μm 2 according to their measured resistances. We conducted most of the electrical measurements in a liquid-helium bath at 4 K, using a dipping probe with a superconducting magnet. A magnetic field was applied parallel to the long axes of the devices. The current–voltage ( I – V ) characteristics at each magnetic field were fit to the resistively shunted junction model [23] , yielding I m and the normal resistance R n ( Fig. 2d ). Because of the GMR effect, the junction resistance is slightly smaller in the P state than in the AP state. The magnetoresistance ratio is roughly 0.2% in a Ni 0.7 Fe 0.17 Nb 0.13 (2.1 nm)-Ni(3 nm) PSV. 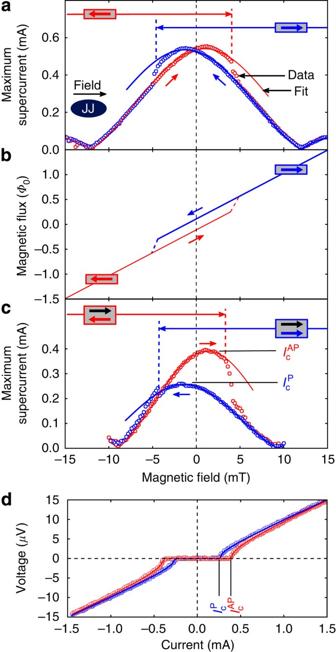Figure 2:Electrical measurement results of S–PSV–S JJs with magnetic field. (a) Maximum supercurrent versus magnetic field of a JJ with zero Ni thickness (dNi≈0) in the PSV barrier structure, Ni0.7Fe0.17Nb0.13(2.1 nm)/Cu(5 nm)/Ni(dNi). The JJ design is a 0.9 μm × 1.8 μm ellipse and the magnetic field is applied along the long axis of the ellipse (inset). (b) Total magnetic flux in the junction versus field inferred from the offsets in the Fraunhofer-like patterns ina. (c) Maximum supercurrentImversus magnetic field of the S–PSV–S device withdNi=1 nm. The JJ design is a 1.2 μm × 2.4 μm ellipse. (d) Current versus voltage of the device used incmeasured at the magnetic field giving the peakImfor each state. The measurement temperature is 4 K.andare the critical currents with the P and AP magnetization states of the PSV barrier, respectively. Symbols are measured data and lines are fits. The magnetization states are labelled by coloured and black arrows in the illustrated boxes above the plots for the Ni0.7Fe0.17Nb0.13and the Ni layers, respectively. Figure 2: Electrical measurement results of S – PSV – S JJs with magnetic field. ( a ) Maximum supercurrent versus magnetic field of a JJ with zero Ni thickness ( d Ni ≈0) in the PSV barrier structure, Ni 0.7 Fe 0.17 Nb 0.13 (2.1 nm)/Cu(5 nm)/Ni( d Ni ). The JJ design is a 0.9 μm × 1.8 μm ellipse and the magnetic field is applied along the long axis of the ellipse (inset). ( b ) Total magnetic flux in the junction versus field inferred from the offsets in the Fraunhofer-like patterns in a . ( c ) Maximum supercurrent I m versus magnetic field of the S–PSV–S device with d Ni =1 nm. The JJ design is a 1.2 μm × 2.4 μm ellipse. ( d ) Current versus voltage of the device used in c measured at the magnetic field giving the peak I m for each state. The measurement temperature is 4 K. and are the critical currents with the P and AP magnetization states of the PSV barrier, respectively. Symbols are measured data and lines are fits. The magnetization states are labelled by coloured and black arrows in the illustrated boxes above the plots for the Ni 0.7 Fe 0.17 Nb 0.13 and the Ni layers, respectively. Full size image Magnetic switching of an S–F–S JJ Figure 2a shows the measured I m ( H ) of an S–F–S JJ with the magnetic field swept in both directions to see the magnetic hysteresis. (Technically, it is an S–PSV–S junction with an ultra-thin Ni layer thickness, d Ni <0.1 nm; because of an error in shutter operation, a trace amount of Ni less than a monolayer in thickness was deposited.) For this control sample, the Ni is so thin that it has no measureable moment and the barrier is effectively a single magnetic layer. From the positive field limit to roughly −5 mT, the magnetic state of the device stays close to a fully magnetized, single-domain state, and the I m ( H ) characteristic follows a smooth Fraunhofer-like pattern. Excluding the abrupt changes, where the Ni 0.7 Fe 0.17 Nb 0.13 layer switches, these data can be fit by conventional theory with a horizontal shift to account for the offsets due to the net self-field of the ferromagnetic state within the barrier. To fit our data, we use I m = I c |2 J 1 ( πΦ / Φ 0 )/( πΦ / Φ 0 )|, for a circular or elliptical junction, [23] where J 1 is a Bessel function of the first kind. Φ and Φ 0 are the magnetic flux through the junction and the flux quantum, respectively. As I m ( H ) is sensitive to junction shape, J c uniformity, field uniformity and so on, this simple formula is not expected to provide a perfect fit at high fields. However, it works reasonably well for the main lobes of both PSV states. Such undistorted shapes as well as the nodes with I m ≈0 indicate no trapped flux in the junction. Each pattern is shifted in the direction opposite to the Ni 0.7 Fe 0.17 Nb 0.13 magnetization, as expected. The total magnetic flux in the junction can be inferred from the added or subtracted offsets at the switching fields on top of the linear increase with applied field ( Fig. 2b ). Such hysteretic magnetization loops in JJs with a magnetic barrier have been previously reported and understood well [13] , [27] . The critical current I c for each magnetization state is given by the main peak of each I m ( H ) for that state. The critical currents for each state are identical for this S–F–S junction, indicating no change in the Josephson coupling ( I c or J c ), because the magnetization of the single F layer in the barrier is simply changing direction. Magnetic switching of S–PSV–S JJs When adding a thicker Ni layer to form a PSV barrier, we find a different I c for each magnetic state of the S–PSV–S junction ( Fig. 2c ). We magnetized the Ni layer to near-saturation with μ 0 H ≈200 mT and removed the resulting trapped flux in the superconducting Nb by raising the sample temperature above 9 K. The sample temperature was then lowered to 4 K and I m was measured over a ±10 mT field range. The abrupt transitions of I m ( H ) indicate that the reversal of the Ni 0.7 Fe 0.17 Nb 0.13 layer begins at −4 mT in one direction and at +3 mT in the other direction. The two distinctly different peak values, and for P and AP states, respectively, definitively demonstrate that the Josephson coupling can be controllably modulated by the exchange field in a PSV and that our measurements have successfully differentiated the Josephson coupling from the remanent-field effect. The remanent-field effect is significant for junction areas down to ≈1 μm 2 in our devices, despite the use of weak and thin ferromagnets. However, any nanoscale device designed to exploit the remanent-field effect will suffer from a small I m modulation, because a reduced total magnetic moment and an increased demagnetizing field in the barrier result in a smaller magnetic flux trapped in the junction. The change in I c , , by the exchange field persists in our smallest junctions as well as in the largest ones ( Fig. 3a ). These results, for the first time, demonstrate the possibility of switchable nanoscale superconducting devices that may enable high-density integration for practical cryogenic memory. 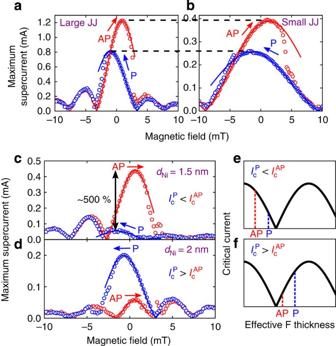Figure 3: Effects of different device areas and Ni thicknesses. Maximum supercurrent versus magnetic field characteristics of various S–PSV–S JJs are compared. (a,b) The effects of different junction areas. The actual areas are estimated to be (a) 2.6 μm2and (b) 0.78 μm2, based on theRnAeff≈ 8.0 mΩ μm2. The JJ designs are (a) 1.6 μm × 3.2 μm and (b) 1.2 μm × 2.4 μm ellipses. The Ni thickness is 1 nm for both JJs. (c,d) Very largeΔIcwith opposite signs for two different Ni thicknesses (c) 1.5 nm and (d) 2 nm. As designed, both JJs are 1.4 μm × 2.8 μm ellipses. The symbols and the curves represent data and fits, respectively. (e,f) Illustrations of the origin of the differentΔIcincandd, respectively. Effective F thickness means the Ni thickness that would result in the same phase shift in the PSV. The decay inIcis ignored for simplicity. A P or AP state results in an increased or decreased phase (blue or red dashed line) relative to that given by the Ni thickness only. The measurement temperature is 4 K. Figure 3: Effects of different device areas and Ni thicknesses. Maximum supercurrent versus magnetic field characteristics of various S–PSV–S JJs are compared. ( a , b ) The effects of different junction areas. The actual areas are estimated to be ( a ) 2.6 μm 2 and ( b ) 0.78 μm 2 , based on the R n A eff ≈ 8.0 mΩ μm 2 . The JJ designs are ( a ) 1.6 μm × 3.2 μm and ( b ) 1.2 μm × 2.4 μm ellipses. The Ni thickness is 1 nm for both JJs. ( c , d ) Very large ΔI c with opposite signs for two different Ni thicknesses ( c ) 1.5 nm and ( d ) 2 nm. As designed, both JJs are 1.4 μm × 2.8 μm ellipses. The symbols and the curves represent data and fits, respectively. ( e , f ) Illustrations of the origin of the different ΔI c in c and d , respectively. Effective F thickness means the Ni thickness that would result in the same phase shift in the PSV. The decay in I c is ignored for simplicity. A P or AP state results in an increased or decreased phase (blue or red dashed line) relative to that given by the Ni thickness only. The measurement temperature is 4 K. Full size image Analysis of junctions with a range of d Ni provides further insight into the exchange-field effect in S–PSV–S devices. The results presented in Figs 2c and 3a,b show that , or ΔI c <0. As the exchange-field effect produces a phase shift of the pair wavefunction, if the thickness of one of the F layers is varied, then ΔI c will oscillate as well, including sign changes. That is, the slope of a sinusoidal function oscillates as well as the function itself. Figure 3e,f illustrate this point with the PSV barrier structure projected to a single F, that adds a phase proportional to an effective F thickness; here we do not take account of the phase decoherence that only leads to an overall decay in I c . The phase shift, hence the effective F thickness, is larger for the P state than for the AP state, and depending on the slope at the effective thickness of the hard layer, the sign of ΔI c can be either positive or negative. We demonstrated this behaviour by fabricating and measuring JJs with different Ni thicknesses in the PSV barrier. As shown in Figs 3c,d , we found two Ni thicknesses, d Ni =1.5 nm and 2.0 nm, that produced very large ΔI c with opposite signs. Such a sign change in ΔI c is a signature of the exchange-field effect, which has not been observed to date, and shows how prominent changes in superconducting properties can result from the competition between superconducting and magnetic orders. A more complete trend has been obtained by varying d Ni . With 0< d Ni <4 nm, we obtained a characteristic voltage V c ≡ I c R n , for each state, and , which showed different oscillatory trends ( Fig. 4 ). We can readily understand that ΔV c also oscillates and changes sign. Each V c ( d Ni ) has a typical trend observed in S–F–S JJs [28] , [29] with different offsets in d Ni between the P and the AP states. Such different thickness offsets, and , originate from the added opposite phases with the two different magnetization orientations of the Ni 0.7 Fe 0.17 Nb 0.13 layer. 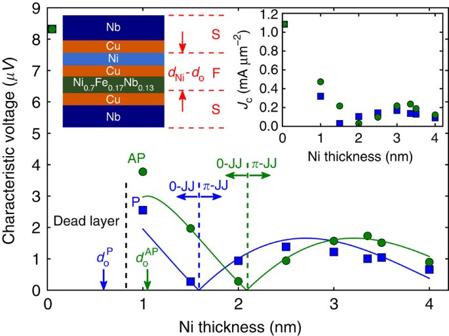Figure 4:Characteristic voltageVcversus Ni thickness of S-PSV-S devices. The PSV structures are Ni0.7Fe0.17Nb0.13(2.1 nm)/Cu(5 nm)/Ni(dNi) with varyingdNi. Symbols and solid lines are data and fits, respectively. The measurement temperature is 4 K. P and AP states are indicated by blue squares and green circles, respectively. EachVcdatum is an average for a few JJ samples. FordNi<3 nm, eachVcdatum is an average for either three or four devices, resulting in an error bar comparable to or smaller than the marker size (the standard error of the meanIc≤20 % of the meanIc). FordNi≥3 nm, the sample size is 1. Left inset: device multilayer structure and its equivalent S–F–S structure as an approximation. Right inset: critical current densityJc(given byVc/RnAeff) versus Ni thickness. Consequently, both and can be described by an S–F–S theory for the clean limit with different and , respectively [30] : Figure 4: Characteristic voltage V c versus Ni thickness of S-PSV-S devices. The PSV structures are Ni 0.7 Fe 0.17 Nb 0.13 (2.1 nm)/Cu(5 nm)/Ni( d Ni ) with varying d Ni . Symbols and solid lines are data and fits, respectively. The measurement temperature is 4 K. P and AP states are indicated by blue squares and green circles, respectively. Each V c datum is an average for a few JJ samples. For d Ni <3 nm, each V c datum is an average for either three or four devices, resulting in an error bar comparable to or smaller than the marker size (the standard error of the mean I c ≤20 % of the mean I c ). For d Ni ≥3 nm, the sample size is 1. Left inset: device multilayer structure and its equivalent S–F–S structure as an approximation. Right inset: critical current density J c (given by V c / R n A eff ) versus Ni thickness. Full size image In (1), Δ is the order parameter of the superconducting electrodes, T is the temperature and α ≡2 E ex ( d Ni − d 0 )/ ℏ ν F with the exchange energy E ex of Ni and the Fermi velocity v F . We note that Δ represents a reduced order parameter at the interfaces of Ni in this simplified model (S/Ni/S). The use of this quasi-classical theory should be appropriate for Ni thicknesses between several atomic layers and the electron mean free path (for example, ~5 nm from Blum et al. [31] ) and results in good fits to the measured V c data for d Ni ≥1.5 nm (see Fig. 4 ). d o includes the thin effective dead layer d dead in Ni; we obtained , that is, a dead layer of 0.4 nm at each Ni/Cu interface. This is comparable to the commonly observed magnetic dead layers in F/N structures [32] and is roughly consistent with our measured saturation magnetization versus thickness of Ni without a Ni 0.7 Fe 0.17 Nb 0.13 layer. We expect a non-oscillatory decay of V c and zero ΔV c within the dead layer if the ferromagnetism is completely suppressed [33] , [34] . However, the exchange-field effect, and hence non-zero ΔV c , may gradually appear around d dead . The V c (or J c ) oscillating period of 2.6 nm and the characteristic length given by ℏ ν F /2 E ex =1 nm roughly agree with past reports regarding simple Nb/Ni/Nb JJs [31] , [33] , [34] . The superconducting order is much reduced in a PSV as indicated by the fitted Δ (≈50 μV) that is smaller than that of Nb by more than an order of magnitude. This originates mostly from strong pair decoherence in Ni 0.7 Fe 0.17 Nb 0.13 , which we separately confirmed by observing the steep decay of J c with its thickness. However, because decohered pairs are shunted by supercurrent and thus excluded from our I c measurement, the fidelity of the supercurrent oscillation is not compromised as evidenced by the near-extinction of V c at the 0- π transition nodes. Such a filtering effect does not exist in non-superconducting spintronic devices in which all the carriers contribute to the measured current and decoherence degrades the measurement fidelity in general. Possibilities of new device applications follow from this exchange-field effect. The node in each V c ( d Ni ) in Fig. 4 represents the transition of the zero-field JJ ground state from 0 to π in phase difference [4] , [5] , [28] , [29] . Such transitions occur at different d Ni values of 1.6 nm and 2.1 nm for the P and AP states, respectively, which implies that JJs with 1.6 nm < d Ni <2.1 nm are phase-switchable devices. Phase-shifting elements are novel components of superconducting digital and qubit electonics [35] , [36] , [37] , [38] . Among the different device types, S–F–S JJs are often considered the most promising architecture for a π -phase shifter due to their non-volatility and small size [38] . For example, the proposed elimination of the superconducting loops in some rapid single-flux quantum logic components by use of π -JJs [36] has been experimentally demonstrated with S–F–S devices [39] . It will be interesting to see what kind of novel future electronics will be conceived and realized with the added capability of in situ , non-volatile phase switching offered by S–PSV–S JJs. Regarding the cryogenic memory application of these devices, the near-extinction of I c at a 0- π transition is an important feature, as it facilitates reliable discrimination of the information stored in the PSV states. A large bias-current margin for discriminating between the low and high I c states in a cryogenic memory based on single JJs will be essential in overcoming device-parameter spreads in highly integrated circuits. A useful metric for this margin is the relative change in I c , | ΔI c |/(the lesser of and ) ≈500 % for d Ni =1.5 nm ( Fig. 3c ). This is well beyond a typical GMR ratio of a spin valve (<10%) and is comparable to the best present-day tunnelling magnetoresistance ratios of ≈600 % at room temperature and ≈1,100 % at 4.2 K [40] . Determining the fundamental limit to that margin may require investigation of higher-harmonic Josephson currents, I m sin nθ ( n =2, 3, …), which may remain finite even at the 0- π transition node [30] , [33] , [41] . Such a large margin may allow reading memory states with a very low error rate. In addition, the use of Josephson energy as a memory parameter implies the inherent compatibility with SFQ (single flux quantum) electronics and may be probed by an SFQ. As an SFQ signal is ballistic with a speed of light and only dissipates very low energy in a junction, memory elements based on switchable Josephson energy may prove to be a way to overcome the speed and power limitation of conventional charge- or resistance-based devices. How to cite this article: Baek, B. et al. Hybrid superconducting-magnetic memory device using competing order parameters. Nat. Commun. 5:3888 doi: 10.1038/ncomms4888 (2014).